Terahertz underdamped vibrational motion governs protein-ligand binding in solution Low-frequency collective vibrational modes in proteins have been proposed as being responsible for efficiently directing biochemical reactions and biological energy transport. However, evidence of the existence of delocalized vibrational modes is scarce and proof of their involvement in biological function absent. Here we apply extremely sensitive femtosecond optical Kerr-effect spectroscopy to study the depolarized Raman spectra of lysozyme and its complex with the inhibitor triacetylchitotriose in solution. Underdamped delocalized vibrational modes in the terahertz frequency domain are identified and shown to blue-shift and strengthen upon inhibitor binding. This demonstrates that the ligand-binding coordinate in proteins is underdamped and not simply solvent-controlled as previously assumed. The presence of such underdamped delocalized modes in proteins may have significant implications for the understanding of the efficiency of ligand binding and protein–molecule interactions, and has wider implications for biochemical reactivity and biological function. When a ligand binds to a protein, which can result in large conformational changes and domain movements, there are more subtle changes within the protein that can give rise to altered protein flexibility and that are potentially biologically important. However, there is considerable variation in the nature and even direction of such changes. For example, several proteins exhibit increased flexibility in the protein–ligand complex, which has been observed using neutron scattering [1] and NMR studies [2] , [3] , whereas other experiments have observed a stiffening and reduction in flexibility [4] . These changes are likely to influence the affinity of binding and the stability of the protein–ligand complex. Protein flexibility is considered to be dependent on low-frequency (<100 cm −1 ; <3 THz) vibrational modes and the presence of additional intermolecular interactions between the ligand and the protein can lead to changes in the vibrational spectrum [5] . Previous theoretical studies have carried out normal-mode calculations on a range of proteins in order to determine the frequency and character of these vibrational modes [6] . For example, in the enzyme lysozyme, this has led to the identification of a 3–4 cm −1 (~100 GHz) highly delocalized hinge-bending mode that opens and closes the binding cleft [7] , [8] . However, in aqueous solution, such very-low-frequency modes are likely to be heavily overdamped and hence impossible to detect using vibrational spectroscopy [9] . Nevertheless, such very-low-frequency overdamped modes are likely to play an important role in flexibility and will affect the free energy of binding [5] . In contrast, there have been suggestions that terahertz-frequency underdamped collective modes of the protein may direct the system along the correct path on a highly complex potential-energy surface [10] , and may be responsible for the low-loss transport of energy through the protein [11] , which may facilitate biological function through phonon-like modes [12] . Theoretical models of enzymes have indeed suggested that concerted conformational fluctuations on a femtosecond to picosecond timescale promote catalysis by coupling to the reaction coordinate [13] , [14] , [15] , [16] . This model is also supported by experiments in which the direct excitation of terahertz-frequency modes with far-infrared light was shown to enhance the reaction rates in proteins [17] . However, the role of terahertz-frequency vibrational modes in mediating efficient protein-ligand binding and biochemical reactions in general is not known. Several groups have attempted to measure the vibrational spectra of proteins in the terahertz range directly in the hope of finding peaks that could then be assigned to biochemically relevant motions in the protein. Femtosecond pump-probe experiments on proteins with light-absorbing chromophores, such as heme proteins [18] , [19] and photosynthetic light-harvesting proteins [20] , [21] , have shown that some modes in the terahertz range are in fact underdamped. However, these underdamped motions were restricted to Franck–Condon active vibrational modes of chromophores and any involvement in ligand binding or catalysis could not be established. Far-infrared and terahertz time-domain spectroscopy (THz-TDS) have been used to study proteins in solution but have been largely unsuccessful due to the very large absorption by liquid water [22] . Although recent THz-TDS experiments on lysozyme crystals have successfully identified underdamped delocalized vibrational modes in the terahertz range [23] , the crystal packing and hydration level modify the protein dynamics, and it remains impossible to show the biochemical relevance of such modes. Inelastic neutron scattering [24] , [25] and spontaneous Raman scattering [26] , [27] , [28] , [29] have been used to study lysozyme in solution and do not suffer from water absorption. However, these techniques become unreliable at low frequencies (<1 THz) due to the very strong Rayleigh peak from elastic scattering, and again it has not been possible to assign biochemical relevance to any peaks observed. Femtosecond optical Kerr-effect (OKE) spectroscopy allows the measurement of the depolarized Raman spectrum in the time domain. Although in principle OKE spectroscopy measures the same signal as spontaneous Raman scattering, in practice OKE is superior at low frequencies, as it does not suffer from a large Rayleigh peak [30] . The OKE signal arises from orientational motions that in proteins include the librational motions of amino-acid side chains. It has been shown previously that OKE is sensitive to protein structural motifs that appear in the terahertz region [31] , [32] , [33] . Here, we show OKE spectra of an enzyme in aqueous solution and, to investigate the biochemical relevance of any spectral features found, we compare the OKE spectra of the enzyme with and without a bound inhibitor [34] , [35] . Through developments that yield an improvement in the signal-to-noise ratio of several orders of magnitude, we achieved a much wider spectral bandwidth from below a gigahertz up to tens of terahertz (0.03–1000, cm −1 ), providing continuous high-fidelity coverage that no other technique can match [36] , [37] . This advantage means that small changes in a particular spectral region, which might appear as a simple amplitude change when observed within a narrow frequency range, can be identified and interpreted correctly. The dramatically improved signal-to-noise ratio hence allows the reliable detection of small changes induced by biochemical means. We can therefore probe the functional dynamics of ligand binding and here we apply it to lysozyme as a prototypical small highly soluble enzyme. Lysozyme cleaves the β-(1→4) glycosidic bond between an N -acetylglucosamine sugar (NAG) and an N -acetylmuramic acid sugar or between two NAG units in the poly-NAG chitin. However, N,N′,N″ -triacetylchitotriose (NAG 3 ) is not cleaved but binds to lysozyme with high affinity and is an effective enzyme inhibitor (see Supplementary Note 1 ). In the OKE spectra of lysozyme solutions, we identify a terahertz-frequency underdamped delocalized vibrational mode that blue shifts and increases in intensity upon binding of NAG 3 . OKE spectroscopy An OKE spectrum for hen egg-white lysozyme (15 mM in sodium acetate buffer, pH 5.4) was obtained at 298 K ( Fig. 1a ). Very similar results were obtained when the enzyme was dissolved in water and in Tris buffer at pH 8 (data not shown). Acetate buffer alone gives a very weak OKE signal and hence, at the concentration used (0.1 M), the spectrum of the buffer was indistinguishable from that of water. The latter is relatively weak and well known [38] . Subtracting the solvent spectrum from the spectrum of the lysozyme solution yields a difference spectrum that is predominantly due to the solvated protein ( Fig. 1a ). 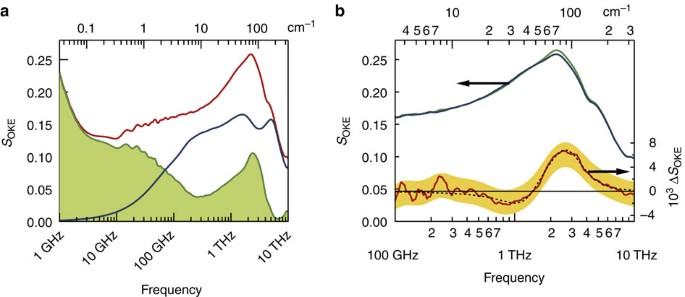Figure 1: OKE spectra for lysozyme solution. (a) Hen egg white lysozyme solution (red) and buffer solution (blue). The protein spectrum has a pronounced peak that the simple difference (green) reveals to have a narrow peak at 2.8 THz accompanied by a broad shoulder around 1 THz. Below 5 GHz is the edge of the protein orientational diffusion band and the additional broader peak above this can be explained as the contribution of the restricted diffusion of water in the protein hydration layer. (b) Terahertz region of the OKE (solvent-subtracted) spectra for lysozyme only (blue) and in a complex with triacetylchitotriose (green). The difference spectrum highlights the increase in intensity at ca. 3 THz with a weaker reduction in intensity at ca. 1 THz. The yellow region is the estimated uncertainty in the difference spectrum based on the repeatability of the measurements. The dashed trace is a fit by two brownian oscillators. Figure 1: OKE spectra for lysozyme solution. ( a ) Hen egg white lysozyme solution (red) and buffer solution (blue). The protein spectrum has a pronounced peak that the simple difference (green) reveals to have a narrow peak at 2.8 THz accompanied by a broad shoulder around 1 THz. Below 5 GHz is the edge of the protein orientational diffusion band and the additional broader peak above this can be explained as the contribution of the restricted diffusion of water in the protein hydration layer. ( b ) Terahertz region of the OKE (solvent-subtracted) spectra for lysozyme only (blue) and in a complex with triacetylchitotriose (green). The difference spectrum highlights the increase in intensity at ca. 3 THz with a weaker reduction in intensity at ca. 1 THz. The yellow region is the estimated uncertainty in the difference spectrum based on the repeatability of the measurements. The dashed trace is a fit by two brownian oscillators. Full size image For proteins, even small globular ones such as lysozyme, the large moment of inertia means that the molecular orientational diffusion has a timescale of a few megahertz [39] and only the high-frequency tail can be seen in Fig. 1a below ~5 GHz. This feature was unreliable, suggesting that these highly viscous solutions do not fully relax within the timescale of the experiments. A weaker shoulder that appears between 10 and 200 GHz can be explained as ‘slow’ water diffusing within the protein hydration layer [28] , [40] . The outstanding feature in the solvated-protein spectrum is a distinctive peak just above 2 THz with a broad low-frequency shoulder. This feature can be fitted by a pair of brownian oscillators (see methods and Supplementary Fig. 1 ), yielding the parameters ω 0 =1.15 THz and γ =0.52 THz for the broad shoulder and ω 0 =2.80 THz and γ =1.24 THz for the narrow peak. As the damping γ is less than the frequency ω 0 , this implies that the vibrational mode involves an underdamped oscillator. The OKE spectra of simple molecular liquids generally give a pronounced peak at 1–3 THz that arises from librations [30] , that is, oscillatory small-angle rotations of the whole molecule in the solvent ‘cage’. For larger molecules such as proteins, the terahertz spectrum is due to the intramolecular flexibility that allows torsional and bending motions of the protein backbone with consequent partial rotations (librations) [41] and torsions [42] of the side chains. If the solvated-protein spectrum in the terahertz range were due to multiple localized modes, one would expect an inhomogeneous gaussian distribution of local-mode frequencies—reflecting different local masses and forces—giving rise to a broad overdamped spectrum. This is not observed. An alternative explanation for the observed signal is librations of individual amino acids. Orientational motions of those moieties with the highest polarizability anisotropy would produce the largest OKE signals. Hence the tryptophan residues, with their planar fused-aromatic indole group, are expected to make the strongest contributions to the OKE spectrum of lysozyme. In Fig. 2 , the OKE spectrum of tryptophan in solution is shown at the same concentration as used for the lysozyme spectrum. This reveals a broad librational band at ~2 THz that is more than an order of magnitude weaker than the sharp 2.8 THz peak seen in lysozyme. Previous OKE studies of styrene and polystyrene have shown a reduction in the librational band strength by a factor of three upon polymerization [41] . Thus, the contribution of each individual tryptophan residue to the lysozyme spectrum is expected to be nearly two orders of magnitude weaker than the sharp 2.8 THz peak. 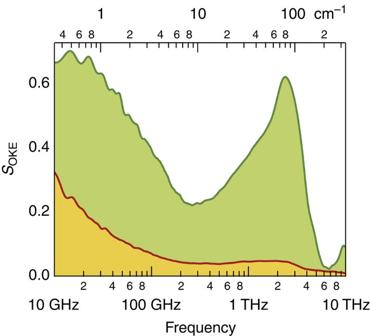Figure 2: Comparison of the OKE spectra for lysozyme and tryptophan. Both spectra were taken in aqueous solution at a concentration of 15 mM with the solvent spectrum subtracted. The tryptophan solution with the solvent subtracted (red) reveals a weak spectrum compared to the lysozyme spectrum (green). The increase at low frequency (<100 GHz) in the tryptophan spectrum is due to single-molecule orientational diffusion, which is absent for residues of a protein. Figure 2: Comparison of the OKE spectra for lysozyme and tryptophan. Both spectra were taken in aqueous solution at a concentration of 15 mM with the solvent spectrum subtracted. The tryptophan solution with the solvent subtracted (red) reveals a weak spectrum compared to the lysozyme spectrum (green). The increase at low frequency (<100 GHz) in the tryptophan spectrum is due to single-molecule orientational diffusion, which is absent for residues of a protein. Full size image Having discounted the above possible explanations, the sharp terahertz peak observed appears to correspond to a single or a small number of delocalized modes involving motions of many residues. The number of residues involved in such motions is difficult to estimate, as the strength of the contribution of the individual amino-acid residues to the OKE signal is unknown. However, based solely on the measurements shown in Fig. 2 , one can estimate that the delocalized mode is likely to involve at the very least a dozen residues. OKE spectra were then obtained after addition of the lysozyme inhibitor NAG 3 at a protein-to-saccharide molar ratio of 1:1. Measurements for a 15 mM solution of NAG 3 alone showed that the weakly polarizable saccharide makes no measurable contribution. However, the OKE spectrum for lysozyme+NAG 3 shows a pronounced increase in intensity at around 3 THz ( Fig. 1b ). The difference spectrum shows an undulation, comprising an increase in intensity on the higher frequency side of the sharp lysozyme peak, accompanied by a weaker but significant decrease in intensity around 1 THz. From the broad bandwidth of our OKE measurement, it is evident that the spectrum at lower and higher frequencies is unperturbed. A simple interpretation of the undulation feature in the difference spectrum would be of a band shift from 1 to 3 THz. However, for OKE spectra, a band shift in isolation would (as shown in methods and Fig. 3 ) give rise to a negative peak much larger in amplitude than the positive peak whereas here we see the converse. The OKE signal is proportional to the product of the polarizability of the vibrational modes and the vibrational density of states (VDoS). However, the overall VDoS cannot increase in this experiment since the OKE signal from NAG 3 is immeasurably small at the concentration used. Therefore, the anomalous strength of the peak at ~3 THz must be caused by an increase in the polarizability of the mode. This polarizability enhancement is therefore additional to any simple shift from 1 to 3 THz. 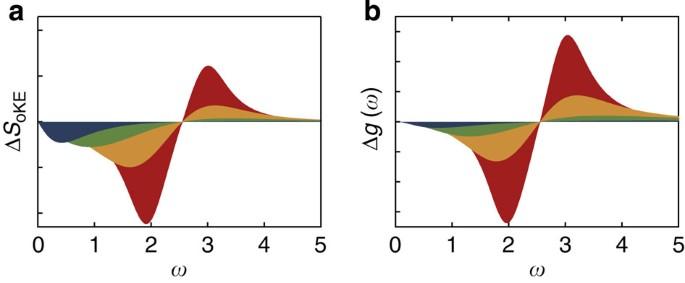Figure 3: Effect of a band shift in the Brownian oscillator model. (a) The change in OKE response ΔSOKEfrom equation (5), and (b) the corresponding change in VDoS Δgfrom equation (6), for the difference signal resulting from a brownian oscillator mode shifting fromω0=2 toω0=3. The damping is set toγ=0.5 (red), 1 (orange), 2 (green) and 4 (blue). Whereas the change in VDoS shows the expected even undulation, the difference OKE signal has a far weaker positive lobe. Figure 3: Effect of a band shift in the Brownian oscillator model. ( a ) The change in OKE response Δ S OKE from equation (5), and ( b ) the corresponding change in VDoS Δ g from equation (6), for the difference signal resulting from a brownian oscillator mode shifting from ω 0 =2 to ω 0 =3. The damping is set to γ =0.5 (red), 1 (orange), 2 (green) and 4 (blue). Whereas the change in VDoS shows the expected even undulation, the difference OKE signal has a far weaker positive lobe. Full size image The difference spectrum can be fitted by a pair of brownian oscillators ( Fig. 1b and Supplementary Fig. 2 ) yielding the parameters ω 0 =1.29 THz, γ =0.64 THz for the negative mode and ω 0 =2.89 THz, γ =1.38 THz for the positive mode. The amplitude of the positive mode is 7.5 times greater than that of the negative mode and since the damping factor γ is less than ω 0 , the mode is significantly underdamped. The undulating difference band is not inhomogeneously broadened into an overdamped lineshape. This implies that it cannot be caused by the sum of many small changes in many local modes. The amplitude of the undulation at 3 THz is 6% of the protein-only spectrum at this frequency, which (based on the relative strength of the OKE signal for tryptophan) rules out that the undulation is caused by the change in environment of a single residue. Thus, the data prove that the undulation is caused by a delocalized mode of the protein blue-shifting accompanied by an increase in polarizability. Molecular dynamics simulations Molecular dynamics simulations were carried out for lysozyme, with and without bound NAG 3 (see Supplementary Note 2 and Supplementary Tables 1–4 for details and additional results), with the principal aim of characterizing the motions around 3 THz, that is, on a timescale of a few hundred femtoseconds. Fourier filtering [43] enabled us to analyse the motions in selected frequency windows. The root mean square fluctuations (RMSFs) of atomic positions for the unfiltered trajectories, which include all frequencies, show the expected pattern: surface residues are more mobile than residues in the core and side chains are more mobile than the backbone ( Fig. 4a ). The outermost sugar ring of NAG 3 , which is exposed to bulk solvent, is much more mobile than the two inner rings, which are more deeply buried in the binding cleft. Analysis of the motions in the 1.5–3.5 THz window shows a distinctly different pattern ( Fig. 4b ). There is no longer a ‘cool’ core and a ‘warm’ surface of the protein. Surface loops, which are very mobile overall, have lower mobility in this frequency range, whereas side chains in the core, which are overall rather rigid, have RMSFs comparable to surface side chains. In NAG 3 , the outermost sugar ring now moves less than the inner rings, in contrast to the pattern in the full spectrum. 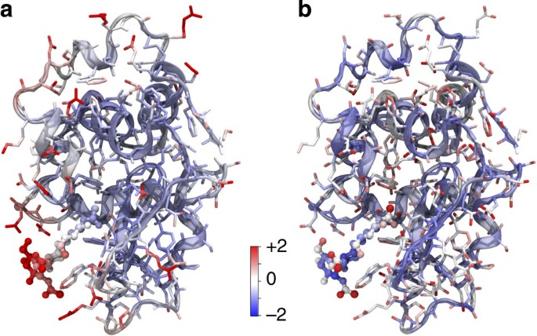Figure 4: Motions of NAG3-bound lysozyme from molecular dynamics. (a) Motions in the full spectral range from unfiltered trajectories. (b) Motions in the 1.5–3.5 THz window from Fourier-filtered trajectories. Atoms (without hydrogens) are coloured by RMSF; the ribbon representation of the backbone is coloured according to the RMSF of the Cα atoms. The colour scale is in units of standard deviations from the mean for the respective frequency range. Figure 4: Motions of NAG 3 -bound lysozyme from molecular dynamics. ( a ) Motions in the full spectral range from unfiltered trajectories. ( b ) Motions in the 1.5–3.5 THz window from Fourier-filtered trajectories. Atoms (without hydrogens) are coloured by RMSF; the ribbon representation of the backbone is coloured according to the RMSF of the Cα atoms. The colour scale is in units of standard deviations from the mean for the respective frequency range. Full size image While side chains on the whole are more mobile than the backbone, both in the full spectrum and the 1.5–3.5 THz window, it is the high RMSFs of the terminal side-chain atoms that stand out in the 1.5–3.5 THz window. Visual inspection of the filtered trajectories revealed that the motions in this frequency range are best described as side-chain librations or hindered rotations about terminal single bonds. These torsional oscillations result in large displacements for the terminal atoms most distant from the backbone; hence they appear ‘hot’ in Fig. 4b . The calculated VDoS (see Supplementary Note 2 and Supplementary Fig. 4 ) has a broad peak at ~2.5 THz, consistent with the experimental spectra. This feature is almost entirely due to contributions from the side chains while the backbone VDoS varies little in the 0.5–10 THz range. This finding agrees with the above characterization of the motions around 2.5 THz as side-chain librations. In comparing the VDoS to the OKE spectrum, it is important to remember that the VDoS includes all internal motions whereas OKE is sensitive only to those that influence the polarizability anisotropy. It is not currently feasible to simulate the OKE spectrum for an entire solvated protein. In an attempt to elucidate the origin of the OKE differences seen upon inhibitor binding, we compared the VDoS and RMSFs for the simulations with and without bound NAG 3 (see Supplementary Note 2 and Supplementary Figs 5 and 6 ). Neither the total VDoS nor its side-chain and backbone contributions differ significantly between the two systems. Similarly, there is no significant difference in the average RMSFs for several frequency windows spanning 0.5–5.5 THz. These results support the interpretation that the difference peak is due to changes in polarizability. Inhibitor binding does not affect the amount of motion overall nor in a specific frequency windows. Many groups have attempted to detect delocalized vibrational modes in proteins in the terahertz range. Raman and THz-TDS spectroscopy of crystalline lysozyme and other proteins shows peaks in the 20–100 cm −1 (~1–3 THz) range [23] , [26] , [27] , [28] , [29] . However, these are very sensitive to crystal packing and hydration levels, and may be associated with phonon modes of the crystal lattice, rather than biologically relevant phenomena. Raman spectroscopy on solutions of lysozyme and other proteins has been able to show that some terahertz bands do exist but again it has been impossible to prove biochemical relevance [26] , [28] , [29] . Here we have shown that the vibrational spectrum of lysozyme in solution exhibits sharp peaks at 1.15 and 2.80 THz corresponding to two underdamped delocalized oscillators that involve the motion of at least a dozen residues in the protein. On addition of the inhibitor NAG 3 a blue shift is observed from 1.29 to 2.89 THz accompanied by an anomalous strengthening of the high frequency mode, which must be due to an increase in the polarizability. As the difference is induced by the binding of NAG 3 to lysozyme, but is not present in the solution of NAG 3 only, the mode must be part of the binding coordinate and hence of biochemical significance. The MD simulations cannot reproduce the OKE spectra of lysozyme or lysozyme+NAG 3 in detail, as they do not include polarizability nor changes in polarizability induced by the binding of NAG 3 . However, they do show that the vibrational motions present in the 1–3 THz range involve delocalized backbone torsional motions and librations of the side chains. The terahertz modes observed here in lysozyme and the ligand-bound complex corresponding to the binding coordinate are significantly underdamped, with the damping parameter γ about half the value of the frequency ω 0 . It seems likely that proteins have evolved such underdamped vibrational motions by providing an interaction site which is pre-organized [44] in order to arrive at the optimal degree of damping for efficient biochemical reactivity and function. OKE experimental details The OKE data were recorded in the standard time-domain step-scan pump-probe configuration and Fourier transformed to obtain the frequency domain depolarized Raman spectrum [30] . A laser oscillator (Coherent Micra) provided ~10 nJ pulses with a nominal wavelength of 800 nm at a repetition rate of 82 MHz. After pre-compensation for group-velocity dispersion in a Homosil prism pair, the beam was split into (90%) pump and (10%) probe beams. A high-speed optical delay line with a resolution of 20 nm (Newport IMS600LM) in the pump beam path controlled the pump-probe relative delay with sub-fs resolution and a maximum delay of 4 ns. The two beams were then co-focused by a 10-cm focal length achromatic lens into the sample. The transmitted probe beam was recollimated by a matching lens and then analysed by the combination of an achromatic quarter-wave retarder, Wollaston prism, and balanced photodiode detector. This combination measures the ellipticity of the polarization of the beam induced by the transient birefringence of the sample (optical-heterodyne detection). The optical material (and hence optical dispersion) in each beam was equalized resulting in a cross-correlation measured in the sample position with a full-width at half-maximum pulse duration of 19–20 fs. To minimize spurious signals from scattered pump light, both pump and probe beams were mechanically chopped at rates of ~ 3 kHz in the ratio of 5:7 with lock-in demodulation at the difference frequency. For the longer-timescale relaxation measurements a second set of data was taken in a similar configuration using a higher pulse energy of typically 1 μJ (depending on the sample) provided by a regeneratively amplified laser (Coherent Legend Elite USX) at a repetition rate of 1 kHz with a pulse duration stretched to ~1 ps. Stretching the pulse enables a higher energy to be used without sample damage or nonlinear effects and reduces the upper bandwidth limit allowing large step size scanning without introducing undersampling artefacts [45] . The time-domain data are numerically transformed to the frequency domain and deconvoluted by dividing by the autocorrelation of the laser pulses. Using this setup, we have been able to measure spectra from 125 MHz to about 10 THz (refs 36 , 37 ). Sample preparation Lysozyme from hen egg white (lyophilized, Fluka) was extensively dialysed in order to remove any impurities that may interfere with the OKE signal. N,N′,N″ -triacetylchitotriose ( ⩾ 95%, Sigma) was used without further purification. The measurements were taken in sodium acetate buffer solution at pH 5.4 (100 mM in deionized and ultrafiltered water) with 250 mg protein in 1 ml buffer solution (corresponding to a concentration of 15 mM). At this pH, the dissociation constant is in the micromolar range so over 95% of NAG 3 should be bound [46] , and the dimerization that occurs at higher pH [47] is avoided. To confirm binding at the concentration used in this work, circular dichroism spectra were recorded (see Supplementary Fig. 3 ). Of the three tryptophan residues in the lysozyme active site (Trp62, Trp63 and Trp108), it is believed that Trp108 dominates the near-UV CD profile [48] . On NAG 3 binding, an increase is observed in the three peaks centred at 281, 287 and 293 nm, which has been assigned to a change in the distance between Trp108 with Glu35 (ref. 48 ). This is in quantitative agreement with the literature showing that there is close to 1:1 binding [49] . OKE response function OKE spectroscopy—sometimes referred to as optical-heterodyne detected Raman-induced Kerr-effect spectroscopy (OHD-RIKES)—measures the depolarized Raman spectrum in the time domain [50] , [51] , [52] . The off-resonant OKE signal is a convolution of pump and probe-laser pulse envelopes with the classical impulse response function [53] , [54] for the appropriate polarizability tensor element α: which can be expressed as the sum of a set of vibrational modes i with coordinates q i : Here, is the polarizability derivative. A model has to be chosen to describe the behaviour of the correlation function; here we will use the brownian oscillator model, which—although limited to homogeneous damping only—has a strong physical basis [53] . In this case, the correlation function has the damped harmonic oscillator form where is the Heaviside step function, γ the damping rate and M the effective mass. Ω is given by where is the undamped (resonant) oscillator frequency. The Fourier transform of is Here, only the imaginary part of the OKE spectrum (and hence of equation (4)) is shown, that is, The relationship between and the vibrational density of states (VDoS) is [55] Hence, OKE does not measure g ( ω ) directly but measures the product of the VDoS and the strength of the coupling with the electromagnetic fields through the Raman effect. Figure 3 shows simulated difference spectra assuming a mode at ω 0 =2 shifts to ω 0 =3, as would be expected in so-called mode hardening. The damping parameter was set to a range of values to represent underdamping ( γ =0.5) through to overdamping ( γ =4). For the OKE response Fig. 3a , it can be seen that in all cases the high-frequency peak is lower in amplitude than the low-frequency peak. However, when the same difference spectra are plotted as a VDoS Fig. 3b , the total density of states (integrated over all positive frequencies) does not change. This is in contrast to the data presented here, where in the OKE spectrum the high-frequency peak is larger. The observed change could imply an increase in the VDoS; however, this is inconsistent with the fact that no OKE signal is seen from the inhibitor alone. The only remaining explanation for the increase in OKE signal is then a change in the coupling factor, that is, an increase in polarizability (specifically, the off-axis terms in the polarizability tensor). How to cite this article: Turton, D. A. et al . Terahertz underdamped vibrational motion governs protein-ligand binding in solution. Nat. Commun. 5:3999 doi: 10.1038/ncomms4999 (2014).